Live-cell multiplane three-dimensional super-resolution optical fluctuation imaging Super-resolution optical fluctuation imaging (SOFI) provides an elegant way of overcoming the diffraction limit in all three spatial dimensions by computing higher-order cumulants of image sequences of blinking fluorophores acquired with a classical widefield microscope. Previously, three-dimensional (3D) SOFI has been demonstrated by sequential imaging of multiple depth positions. Here we introduce a multiplexed imaging scheme for the simultaneous acquisition of multiple focal planes. Using 3D cross-cumulants, we show that the depth sampling can be increased. The simultaneous acquisition of multiple focal planes significantly reduces the acquisition time and thus the photobleaching. We demonstrate multiplane 3D SOFI by imaging fluorescently labelled cells over an imaged volume of up to 65 × 65 × 3.5 μm 3 without depth scanning. In particular, we image the 3D network of mitochondria in fixed C2C12 cells immunostained with Alexa 647 fluorophores and the 3D vimentin structure in living Hela cells expressing the fluorescent protein Dreiklang. A microscope is characterized by its three-dimensional (3D) point spread function (PSF) whose spatial extents determine the resolution in the corresponding spatial dimensions. The image of a single fluorescent molecule essentially corresponds to the PSF centred on the position of the molecule. By sequentially imaging isolated fluorophores, determining their PSF centres and mapping them into a position histogram, localization microscopy can render the sample structure with much finer details than classical fluorescence microscopes [1] , [2] , [3] , [4] , [5] . However, this requires the use of fluorophores that can be photo-switched or -activated stochastically. The characteristic rates of activation and deactivation need to be tuned such that only a sparse subset of molecules is active per exposure and a sufficiently high number of photons can be detected for a precise localization [6] , [7] , [8] . As an alternative to single-molecule localization, super-resolution optical fluctuation imaging (SOFI) achieves super-resolution using higher-order statistics with relaxed requirements on the photo-switching kinetics [9] , [10] . SOFI relies on reversible stochastic and independent intensity fluctuations from fluorophores but tolerates a spatio-temporal overlap of their images, incomplete on-off-switching and moderate visibility of the intensity fluctuations. The method has been successfully demonstrated with semiconductor quantum dots [9] , [11] , organic dyes [12] and fluorescent proteins [13] . With the help of time-correlated single photon counting instrumentation, the stochastic photon emission from single fluorophores and the associated antibunching effect was exploited in combination with a modified SOFI analysis [14] . Recently, SOFI was applied to fluorescence fluctuations induced by stochastic approaches of fluorescence resonance energy transfer pairs [15] , where the energy transfer donor was linked to the structure of interest and the acceptor diffusing in the medium. So far, 3D SOFI has only been demonstrated by stacking sequentially acquired optical sections [13] , [16] . In this paper, we introduce an imaging scheme for the simultaneous acquisition of multiple focal planes. The SOFI analysis can then be performed in 3D to increase the spatial sampling and to improve the resolution in all dimensions. In comparison to the sequential imaging of several depth planes, a parallel multiplane acquisition with a numerically increased depth sampling can significantly reduce the acquisition time and therewith limit the photobleaching of markers. We demonstrate the performance of this approach by imaging mitochondria in fixed cells and the vimentin network in living cells. Multiplane 3D SOFI The most basic implementation of SOFI corresponds to the calculation of the temporal variance of an image sequence of stochastically fluctuating emitters. Owing to the independence of the fluctuations, the signals from different emitters are uncorrelated. In consequence, the variance of the total signal from N emitters is the sum of the variances of every single-emitter signal I i : where i is the index of the emitter, r denotes a pixel location on the detector and t is the time. The signal from a single emitter located at r i corresponds to a sampled and shifted version of the microscope’s PSF U ( r − r i ) with a brightness amplitude ε i times a fluctuation signal s i ( t ) that encodes the temporal fluctuations. The single-emitter variance then reads Obviously, the variance-equivalent PSF is given by the original PSF raised to the power of two. This doubles the spatial frequency support of the corresponding optical transfer function and increases the spatial resolution. Instead of calculating the temporal variance on each pixel separately, the covariance of neighbouring pixels provides an additional advantage as it cancels any uncorrelated noise. Furthermore, by using different combinations of pixel pairs for calculating the covariance, the final image sampling can be increased as the covariance essentially probes the sample in the geometrical mean of the chosen pixel pair ( Fig. 1 ). 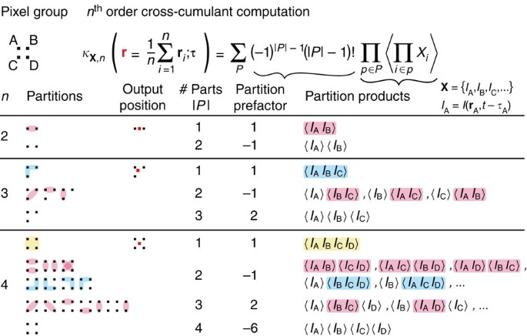Figure 1: Calculation of cross-cumulants. The cross-cumulantκX,nof ordernfor a pixel groupcan be calculated as a sum over all partitions of. Each addend consists of a prefactor depending on the number of parts |P| in the particular partitionPtimes a partition product, which evaluates the partspas a temporally averaged ‹...› product. White, red, blue and yellow backgrounds indicate parts of a partition comprising, respectively, one to four pixels. Figure 1: Calculation of cross-cumulants. The cross-cumulant κ X , n of order n for a pixel group can be calculated as a sum over all partitions of . Each addend consists of a prefactor depending on the number of parts | P | in the particular partition P times a partition product, which evaluates the parts p as a temporally averaged ‹...› product. White, red, blue and yellow backgrounds indicate parts of a partition comprising, respectively, one to four pixels. Full size image Multiplying the PSF with itself for improving the resolution as in the variance and covariance can be generalized to higher orders using cumulants or cross-cumulants [9] , [11] . The second-order cumulant without time lag is equivalent to the variance and the second-order cross-cumulant corresponds to the covariance. An n -th order cumulant or cross-cumulant raises the PSF to the power of n . Cumulants thus provide a mean for resolution enhancement that is ultimately limited by the signal-to-noise ratio (SNR) only. As shown by Dertinger et al . [11] , cross-cumulants among a group of pixel time traces allow to eliminate any noise bias and to increase the pixel grid density, such that the cumulant image resolution is not limited by the effective pixel size. This results in a 3D image with up to n 3 times the original number of pixels for a cumulant order n . Figure 1 illustrates the calculation of cross-cumulants up to the fourth order for pixels { r A , r B , r C , r D } that may differ in any spatial direction including the so far unexploited axial dimension. To maximize the speed and the field-of-view, each dimension of the PSF is oversampled just enough to satisfy Shannon’s sampling theorem [17] and to ensure a correlated signal between the cross-cumulated pixels. For a given spatial sampling distance, the more pixels that are acquired and read simultaneously, the faster the overall image acquisition becomes. It is thus advantageous to use a widefield imaging system with a high pixel-count camera that is sufficiently sensitive and rapid to detect the emitters’ fluorescence fluctuations. In order to fully exploit the resolving power of higher-order cross-cumulants with a balanced image contrast, we applied a simplified linearization [18] . The absolute value of the resulting cumulant image is first deconvolved in 3D using a Lucy-Richardson algorithm. The log-likelihood formulation used in the algorithm is well adapted for cumulants as long as there are no sign changes within a PSF. We then take the n -th root and reconvolve the image with an n -times size-reduced PSF to limit the apparent final resolution to a physically reasonable value given by the support of the cumulant optical transfer function. 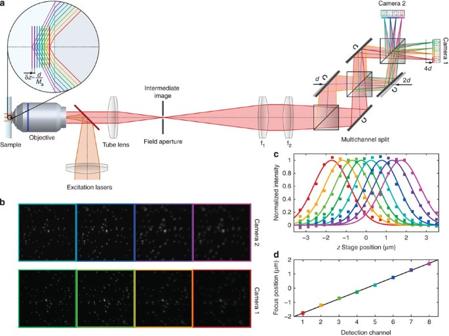Figure 2: Simultaneous detection of multiple focal planes. (a) Multiplane widefield fluorescence microscope. The excitation laser is focused into the aperture of the objective to create a large illumination field. Sample features in several focal planes are imaged simultaneously by two cameras. These focal planes are obtained by splitting the fluorescence into several channels using three 50:50 beam splitter cubes and by introducing path length differencesdand 2dwith the mirrors, as well as 4dwith camera 1 (the grey-shaded element positions would result in a single focal plane detection). The resulting separation between the focal planes in the object space is then approximatelyd/Ma, withMabeing the axial magnification of the system. The images of the focal planes are projected side-by-side on the cameras. A field stop in the intermediate image prevents overlaps between the image frames. (b) Image frames taken with a fluorescent bead sample. (c) Peak brightness in the image frames inbupon scanning the sample plane through the focal channels. (d) Calibration of the focal plane separation by the positions of the brightness maxima inc. Figure 2a outlines a widefield setup for the simultaneous acquisition of multiple focal planes with two cameras. The use of an index-matched immersion objective lens (for example, a water-immersion objective if the sample is in an aqueous environment) minimizes spherical aberrations when imaging thick samples. Three diagonally arranged 50:50 beam splitters behind the lens f 2 split the collected fluorescence into eight separate detection channels. Four mirrors are adjusted to direct the light onto separate areas of the two cameras. By axially shifting two mirrors by a distance d and 2 d as indicated in Fig. 2a and by shifting one camera by a distance 4 d , eight different optical path lengths are achieved with respect to the lens f 2 . Therefore, eight distinct and conjugated depth positions are probed in the sample. The focal plane separation in the object space is then approximately given by d / M a , where M a is the axial magnification (square of the lateral magnification). To comply with Shannon’s sampling theorem, this distance should not exceed half the axial resolution of the imaging system. The field stop has an adjustable rectangular shape and is used to avoid crosstalk between the detection channels. By adding or removing a pair of mirrors and a beam splitter, the number of detection channels can be increased or decreased. Figure 2: Simultaneous detection of multiple focal planes. ( a ) Multiplane widefield fluorescence microscope. The excitation laser is focused into the aperture of the objective to create a large illumination field. Sample features in several focal planes are imaged simultaneously by two cameras. These focal planes are obtained by splitting the fluorescence into several channels using three 50:50 beam splitter cubes and by introducing path length differences d and 2 d with the mirrors, as well as 4 d with camera 1 (the grey-shaded element positions would result in a single focal plane detection). The resulting separation between the focal planes in the object space is then approximately d / M a , with M a being the axial magnification of the system. The images of the focal planes are projected side-by-side on the cameras. A field stop in the intermediate image prevents overlaps between the image frames. ( b ) Image frames taken with a fluorescent bead sample. ( c ) Peak brightness in the image frames in b upon scanning the sample plane through the focal channels. ( d ) Calibration of the focal plane separation by the positions of the brightness maxima in c . Full size image Mitochondria in immunostained fixed cells In view of imaging a deep red emitting organic fluorophore, Alexa 647, we adjusted the distances between the focal planes in the sample to 500 nm ( Fig. 2c,d ). Using a fluorescent bead sample ( Fig. 2b ), we determined the transverse positioning and the mutual distortion of the detection channels for co-registration and measured the full-width-at-half maxima of the PSF in the transverse (320 nm) and axial dimension (1.2 μm). The mutual distortions include the effects of small differences in lateral magnifications and distortions because of non-telecentric and tilted image formation on the camera sensors as well as different wavefront aberrations by the optical elements of the image splitter. We labelled mitochondria by decorating fixed C2C12 cells with antiserum against Tom20, an abundant protein of the outer membrane, and a secondary antibody coupled to Alexa 647. At the imaging conditions, Alexa 647 showed pronounced blinking with an average on time of about 20 ms and an estimated off time of 1–2 s. Taking 5,000 images acquired at 40 frames per second (f.p.s. ), we obtained 3D super-resolved images of mitochondria as shown in Fig. 3 and Supplementary Movie 1 . The simultaneous acquisition of multiple focal planes allowed a volume of 65 × 65 × 3.5 μm 3 to be imaged without scanning. We computed third-order cross-cumulants in order to increase the sampling density threefold in all spatial dimensions. Instead of the original 8 sampling points along the optical axis ( Fig. 3g ), we therefore obtained 22 points, which significantly improves the visibility of structural details in depth ( Fig. 3d–f ). The third-order balanced cumulant image [18] clearly reveals spherical and tubular mitochondrial features ( Fig. 3a,b and d–f ), whereas in the diffraction-limited image those features are barely visible ( Fig. 3c,g ). The strong out-of-focus background is almost completely removed in the 3D SOFI image. As shown in the profiles in Fig. 3h,i , the smallest features resolved in transverse and meridional sections of the image indicate a lateral resolution of about 110 nm and an axial resolution better than 500 nm, which approaches the expected threefold increase in 3D resolution. 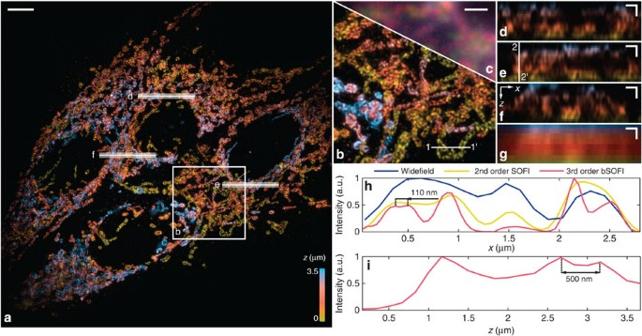Figure 3: Mitochondria stained with Alexa 647 in fixed C2C12 cells. (a) Maximum intensity projection of the third-order balanced SOFI image covering a volume of 65 × 65 × 3.5 μm3. (b) Zoomed region highlighted ina. (c) Diffraction-limited widefield view of the same area asb. (d–f)x–zSections highlighted inaaveraged over 25 pixels alongy. (g) Samex–zsection asffrom diffraction-limited widefield stack. (h)x-Profiles from the cut 1-1′ highlighted inb. (i)z-Profile from the cut 2-2′ highlighted ine. Scale bars: (a) 5 μm (b,c) 2 μm (d–g) 1 μm inxandz. Figure 3: Mitochondria stained with Alexa 647 in fixed C2C12 cells. ( a ) Maximum intensity projection of the third-order balanced SOFI image covering a volume of 65 × 65 × 3.5 μm 3 . ( b ) Zoomed region highlighted in a . ( c ) Diffraction-limited widefield view of the same area as b . ( d – f ) x – z Sections highlighted in a averaged over 25 pixels along y . ( g ) Same x – z section as f from diffraction-limited widefield stack. ( h ) x -Profiles from the cut 1-1′ highlighted in b . ( i ) z -Profile from the cut 2-2′ highlighted in e . Scale bars: ( a ) 5 μm ( b , c ) 2 μm ( d – g ) 1 μm in x and z. Full size image For further comparison, Supplementary Fig. 3 shows the second-order SOFI image without deconvolution and linearization, where we chose a partially saturated image representation to accommodate for the high image contrast. Residual artefacts of the sub-pixel grid are visible around defocused features. Because second-order SOFI improves the resolution only by a factor of approximately (ref. 9 ), third-order balanced SOFI resolves small features significantly better as exemplified by Fig. 3b,h and Supplementary Fig. 3 . Vimentin-Dreiklang-transfected living cells To demonstrate live-cell imaging with short acquisition times, we imaged the vimentin network in living HeLa cells using the reversibly switchable fluorescent protein Dreiklang [19] (cf. Figs 4 and 5 ). Dreiklang possesses three separate but partly overlapping absorption spectra for exciting fluorescence and switching it on and off. This allows for a flexible tuning of photo-switching kinetics and number of photons per switching cycle. We used 405 nm light, which excites in the overlapping absorption bands for switching on and off, to switch Dreiklang at a low on-ratio of about 1%. We used 532 nm light to excite fluorescence well above the absorption maximum in order to avoid switching Dreiklang off at the same time. The distances between the focal planes were then adjusted to 400 nm to account for the shorter wavelength and the resulting reduction in PSF size. The total depth range covered with the eight planes was reduced to 2.8 μm, which was usually too short to cover an entire vimentin network ( Fig. 4a,b ). By increasing the 405 nm illumination intensity, the switching rate of Dreiklang can be increased. We adapted the frame rate so that the exposure time corresponded approximately to the characteristic on-time and changed the fluorescence excitation proportionally in order to determine the maximum acquisition speed yielding a good image quality. With illumination intensities of about 100 W cm −2 at 405 nm and 3 kW cm −2 at 532 nm, the acquisition of about 1,000 frames at 325 f.p.s. was sufficient for a decent SNR in a second-order cross-cumulants analysis ( Fig. 4e,f ). As the total number of emitted photons per fluorophore usually lowers with increasing switching speeds, it is rather preferable to reduce the illumination intensities and accordingly the acquisition speed while keeping motion artefacts small. For Fig. 5 , we reduced the number of planes to four and additionally moved the sample along the axis to cover a total depth of 4 μm in three sequential acquisitions. For a twofold 3D resolution improvement, we evaluated 3,000 images taken at 50 f.p.s. with accordingly reduced illumination intensities of 15 W cm −2 at 405 nm and 450 W cm −2 at 532 nm. 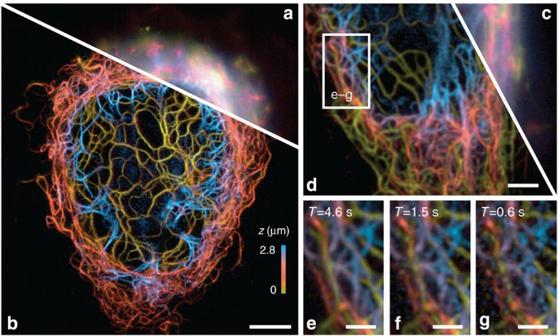Figure 4: Live-cell multiplane SOFI of HeLa cells expressing vimentin-Dreiklang optimized for acquisition speed. Acquisition rates and number of frames: (a,b) 50 f.p.s., 3,000 frames; (c,d) 325 f.p.s., 3,000 frames; (e–g) 325 f.p.s., 1,500, 500 and 200 frames. (a,c) Maximum intensity projection of 8-plane widefield images. (b,d–g) Maximum intensity projection of second-order balanced SOFI. The original eight axial sampling points are complemented by virtual pixels using a 3D second-order cross-cumulant analysis to yield a total of 15. (e–g) Zoomed region highlighted incshowing the resulting second-order balanced SOFI image obtained from 1,500 (4.6 s), 500 (1.5 s) and 200 (0.6 s) frames, respectively, and having the same central time point. For a decent SNR, at least 500 frames seem to be needed. Scale bars: (a,b) 5 μm (c,d) 2 μm (e–g) 1 μm. Figure 4: Live-cell multiplane SOFI of HeLa cells expressing vimentin-Dreiklang optimized for acquisition speed. Acquisition rates and number of frames: ( a , b ) 50 f.p.s., 3,000 frames; ( c , d ) 325 f.p.s., 3,000 frames; ( e – g ) 325 f.p.s., 1,500, 500 and 200 frames. ( a , c ) Maximum intensity projection of 8-plane widefield images. ( b , d – g ) Maximum intensity projection of second-order balanced SOFI. The original eight axial sampling points are complemented by virtual pixels using a 3D second-order cross-cumulant analysis to yield a total of 15. ( e – g ) Zoomed region highlighted in c showing the resulting second-order balanced SOFI image obtained from 1,500 (4.6 s), 500 (1.5 s) and 200 (0.6 s) frames, respectively, and having the same central time point. For a decent SNR, at least 500 frames seem to be needed. Scale bars: ( a , b ) 5 μm ( c , d ) 2 μm ( e – g ) 1 μm. 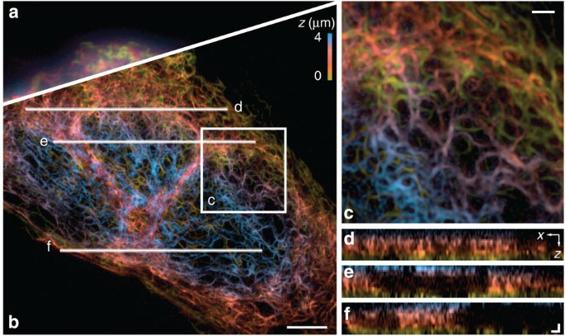Figure 5: Live-cell multiplane SOFI of HeLa cells expressing vimentin-Dreiklang. (a) Maximum intensity projection of widefield images. (b) Maximum intensity projection of second-order balanced SOFI. (c) Zoomed region highlighted inb. (d–f)x–zSections highlighted inb. Scale bars: (a,b) 5 μm (c) 1 μm (d–f) 1 μm inxandz. Full size image Figure 5: Live-cell multiplane SOFI of HeLa cells expressing vimentin-Dreiklang. ( a ) Maximum intensity projection of widefield images. ( b ) Maximum intensity projection of second-order balanced SOFI. ( c ) Zoomed region highlighted in b . ( d – f ) x – z Sections highlighted in b . Scale bars: ( a , b ) 5 μm ( c ) 1 μm ( d – f ) 1 μm in x and z. Full size image For widefield 3D SOFI, it is favourable to acquire multiple depth planes simultaneously. The optimal number of detection channels is limited by the detectable fluctuation signal from the fluorophore and the sensitivity of the detection system. As a guideline, the detected fluctuation amplitude in each channel should at least exceed the read noise amplitude. Using a cross-cumulants analysis of stochastically blinking fluorescent emitters across the individual depth planes, the physically acquired depth planes are supplemented by virtual planes providing a finer depth sampling. As a result, the axial PSF needs not to be n times oversampled as would be the case for axially scanned n -th order 3D SOFI. Accordingly, multiple simultaneously acquired focal planes in combination with 3D cross-cumulants allow for a reduction in the acquisition time and a better exploitation of the available photon budget from the fluorescent markers, particularly if the emitters are prone to bleaching. The resulting contrast of the 3D cross-cumulants is more homogeneous along the optical axis when compared with sequential plane-by-plane 2D cross-cumulants. During sequentially acquired depth sections, the cumulant response of individual emitters might change because of stochasticity resulting in a potentially imbalanced cumulant contrast, which would be problematic for subsequent 3D deconvolution and cumulant balancing (as described in ref. 18 ). As cross-cumulants cancel uncorrelated noise, the image quality is greatly improved. However, auto-fluorescence and/or strongly defocused fluorophores can contribute correlated noise upon photobleaching. Therefore, we minimize photobleaching at best and adjust the sequence length for the data analysis. Some cameras showed correlated read noise, which we attribute to clocking noise upon charge shifting (EMCCD) or row switching (CMOS) at high speed. Therefore, the cameras have been carefully selected for minimizing this correlating bias. The present implementation of a multiplane fluorescence microscope is versatile but susceptible to misalignment of the detection channels because of drift of the components. An integrated image splitter with a minimal number of elements would simplify the alignment and improve the stability. Instead of refractive elements, it is also possible to use a specifically designed 2D grating in combination with glass prisms to generate several depth planes on a single camera [20] . With a wavefront-corrected grating, this concept would enable the use of high-numerical aperture oil-immersion objectives by compensating the spherical aberrations arising from refractive index mismatches. In principle, the resolution in live cells densely stained with Dreiklang could be further improved if the on-time ratio could be lowered, for instance by shifting the switching light to a slightly longer wavelength and thus substantially reduce the on-switching. Alternatively, the fluorescence excitation wavelength could be blue-shifted in order to increase the off-switching while keeping the same on-switching rate. Whereas SOFI can handle multiple markers emitting simultaneously, it is nevertheless beneficial to keep this number reasonably low for improving the visibility of the blinking events. In addition to the improved structural information, SOFI may also provide functional information via a cumulants analysis with different time lags. This enables the quantification of signal fluctuations at different time scales, such as the switching kinetics of the fluorophores and also sample movements. Furthermore, combining the information from several cumulant orders allows to extract spatially resolved molecular state lifetimes, concentrations and fluorescence amplitudes, which may be linked to the surrounding microenvironment [18] . In summary, we introduced a fast and versatile multiplane 3D SOFI concept allowing super-resolved cell imaging in 3D without scanning. We imaged the outer membrane of mitochondria in C2C12 cells as well as the vimentin network of living HeLa cells using an eight-plane detection scheme. Compared with the diffraction-limited image, we demonstrated an up to threefold resolution improvement in all three dimensions in fixed cells and a twofold 3D resolution improvement at acquisition times of a few seconds in living cells. Microscope setup The custom-built microscope system ( Fig. 2a ) comprised a 1.2 numerical aperture × 60 water-immersion objective (UPLSAPO 60XW, Olympus), two diode lasers for excitation and reactivation (MLL-III-635, 800 mW, Roithner Lasertechnik, and iBeam smart, 405 120 mW, Toptica) as well as a green DPSS laser (MLL-FN-532 800 mW, Roithner Lasertechnik), a multiplane splitter with three 50:50 beam splitters (BS013, Thorlabs) and two sCMOS cameras (ORCA Flash 4.0, Hamamatsu). For Alexa 647 imaging, the illumination intensities were adjusted to 2 kW cm −2 at 635 nm (excitation) and 20 W cm −2 at 405 nm (faster reactivation). Dreiklang was switched with 15 W cm −2 at 405 nm and excited with 450 W cm −2 at 532 nm. Dreiklang switching kinetics were measured with the same setup, but with reduced illumination intensities (5.6 W cm −2 at 405 nm, 0.7 W cm −2 at 532 nm) and an additional 365 nm LED epi-illumination with 1.6 W cm −2 (switching on). Data analysis A detailed description of the multiplane SOFI analysis may be found in Supplementary Note 1 with a flowchart given in Supplementary Fig. 1 . In brief, each registered pair of image sequences from consecutive depth channels was divided into 500-frame (Alexa 647) or 100-frame (Dreiklang) sub-sequences and processed with a 3D cross-cumulants analysis using voxel combinations without repetitions ( Supplementary Fig. 2 ) and zero time delays. The frames of one depth sequence were analysed without preprocessing, whereas the frames of the other sequence were co-registered using an affine transformation and bilinear interpolation. The transformation parameters were obtained from a calibration measurement using fluorescent beads. A subsequent fine-tuning of the image registration using a rigid transformation on the measurement data was necessary to correct for residual mechanical drift of the detection optics. From each bi-plane cross-cumulants analysis, only virtual planes and the untransformed physical plane were kept for further processing, because the transformed depth plane contains correlated noise parts in neighbouring pixels introduced by the interpolation. The heterogeneous pixel weights—arising from different responses in the detection channels as well as the the different pixel groups used in the cross-cumulants—were corrected by dividing their respective standard deviations throughout the entire image. Compared with the original SOFI algorithms [11] , [18] suggesting a distance-factor correction by fitting a PSF model that maximizes the image smoothness, this standard-deviation equalization has the advantage of being easier, faster and it seemed more robust with low SNRs, and the different detection responses are automatically corrected. Subsequently, the bi-plane cumulant image blocks are transformed using the previously determined transformation masks in order to have all planes aligned. Finally, the nonlinear response of the cumulant with respect to differences in molecular brightness and blinking was linearized by using a 3D Lucy-Richardson deconvolution, taking the n -th root and reconvolving with an n -times size-reduced PSF. For the display of the z coordinate, we used an ‘isolum’ colourmap compatible with red-green colour perception deficiencies [21] . Cell cultures C2C12 cells were cultured at 37 °C with 5% CO 2 using DMEM high glucose (4.5 g l −1 of glucose), containing 10% fetal bovine serum, 2% HEPES 1 M, 1% MEM Non-Essential Amino Acids Solution (100 × ) and 40 μg ml −1 of Gentamycin (all products were purchased from Life Technologies Corporation). Cells were plated in 35 mm Fluorodish Cell Culture Dish (World Precision Instruments) at roughly 50,000 cells per plate on the day before fixation. HeLa cells were cultured at 37 °C with 5% CO 2 using Minimum Essential Medium Eagle with Earle’s salts, L -glutamine, sodium bicarbonate complemented with 10% fetal bovine serum, 1 × penicillin-streptomycin, 1 × GlutaMAX, 1 × MEM Non-Essential Amino Acids Solution (all products were purchased from Life Technologies). Cells were plated in 4-well Nunc Lab-Tek II Chambered Coverglass (Thermo Fisher Scientific). Immunostaining C2C12 cells were washed three times carefully with PBS and were then incubated for 10 min at room temperature (RT) in 10% neutral buffered formalin solution (4% (w/v) formaldehyde, Sigma-Aldrich) for fixation, followed by washing three times 5 min with PBS. The cells were then incubated for 60 min in TBS containg 0.1% Tween-20 (TBST) with 10% fetal calf serum (FCS) at RT, followed by incubation overnight at 4 °C with a primary antibody for Tom20 (mouse monoclonal, Abcam, ab56783) diluted 1:100 in TBST with 10% FCS. Cells were then washed three times for 5 min with PBS and incubated again at RT for 1–2 h with a secondary antibody (donkey anti-mouse, Alexa Fluo 647), diluted 1:150 in TBST with 10% FCS. After washing the cells three times for 5 min with PBS, a postfixation was performed for 10 min with formalin solution at RT. Before addition of a 1:1 PBS/Glycerol solution, the cells were finally washed again three times for 5 min with PBS. Imaging buffer The Alexa 647 samples were imaged using a buffer containing an oxygen scavenger and a thiol. The solutions were prepared using PBS (Sigma-Aldrich), 0.5 mg ml −1 glucose oxidase (Sigma-Aldrich), 40 μg ml −1 catalase (Sigma-Aldrich), 6.6% (w/v) glucose and 10 mM cysteamine (Sigma-Aldrich). Transfection with vimentin-Dreiklang HeLa cells were transfected using FuGENE 6 transfection reagent (Promega). For each 1.5 cm 2 well, 2 μl Fugene were incubated in 33 μl OptiMEM Reduced-Serum Medium (Life Technologies) during 5 min before the addition of 0.67 μg of the plasmid pMD-Vim-Dreiklang [19] . The solution then stayed 30 min at RT before it was carefully distributed over the cells. Cells were then put back into the incubator and were left overnight before imaging. Determination of Dreiklang switching kinetics In order to determine the appropriate illumination intensities for SOFI measurements, we first determined the switching kinetics of Dreiklang from ensemble experiments with transfected HeLa cells. We implemented an additional 365 nm LED illumination (M365L2 from Thorlabs) to characterize both on- and off-switching of Dreiklang. We used the parallel port as a digital 8-port output to control illumination pulsing and camera synchronization via a Matlab Mex-File [22] . All the switching experiments were carried out on the presented setup using a widefield detection and illumination sources at 365, 405 and 532 nm with 1.6, 5.6 and 0.7 W cm −2 , respectively. A first experiment consisted in a repeated sequence of pulses of 532-405-532-365 nm light to characterize the on-switching ratios of both 405 and 365 nm illuminations ( Supplementary Fig. 4a,b ). The signal plotted in Supplementary Fig. 4a,b corresponds to the background-corrected fluorescence response from a cell transfected with Dreiklang averaged over a thresholded image. The population ratios P 365 /P tot and P 405 /P tot (corrected for bleaching) correspond to the estimated on-ratios of 365 and 405 nm light: The second experiment summarized in Supplementary Fig. 4c,d consisted of a pulsed 365 nm and continuous 405 and 532 nm illumination for extracting the absolute kinetics. The average switch-on and switch-off curves are represented in Supplementary Fig. 4d with the fitted characteristic lifetimes τ on =1/ k off,405 and τ off =1/( k on,365 + k on,405 ). The individual on- and off-switching lifetimes for 365 and 405 nm light at the given intensities can then be estimated as How to cite this article : Geissbuehler, S. et al . Live-cell multiplane three-dimensional super-resolution optical fluctuation imaging. Nat. Commun. 5:5830 doi: 10.1038/ncomms6830 (2014).